Ground tit genome reveals avian adaptation to living at high altitudes in the Tibetan plateau The ground tit ( Parus humilis ) is endemic to the Tibetan plateau. It is a member of family Paridae but it was long thought to be related to the ground jays because of their morphological similarities. Here we present the ground tit’s genome and re-sequence two tits and one ground jay, to clarify this controversially taxonomic status and uncover its genetic adaptations to the Tibetan plateau. Our results show that ground tit groups with two tits and it diverges from them between 7.7 and 9.9 Mya. Compared with other avian genomes, ground tit shows expansion in genes linked to energy metabolism and contractions in genes involved in immune and olfactory perception. We also found positively selected and rapidly evolving genes in hypoxia response and skeletal development. These results indicated that ground tit evolves basic strategies and ‘tit-to-jay’ change for coping with the life in an extreme environment. The Tibetan plateau is the largest high-altitude land mass on the Earth, with an area of 2.3 million km 2 and an average elevation of 4,500 m above sea level [1] . The collision of the Indian subcontinent with the Eurasian plate during the Pliocene caused dramatic changes in the climate of the region, which became drier, colder and windier. Forests were replaced by grasslands, glaciers developed and deserts formed [2] . The cold climate in the Tibetan plateau and the resulting hypoxic conditions created environments that are extremely hostile to most organisms. These harsh conditions caused an unusually strong selection that drove speciation and led to the evolution of many animals that are now well-adapted to a life in the Tibetan plateau [3] . To date we only have a limited understanding of the genetic background of these adaptations. One particularly interesting species endemic to the Tibetan plateau is the ground tit ( Parus humilis , Paridae), also known as Hume’s ground tit and Tibetan ground tit. This is a drab coloured songbird that, unlike other tits, dwells exclusively above the tree line (3,300–5,400 m) on rocky steppes and grasslands of the Tibetan plateau [4] . Previous phylogenetic analysis suggest that the ground tit has evolved from an arboreal ancestor of the genus Parus , the tits [5] . However, in contrast to its closest relatives, the ground tit has a longer and distinctly downward decurved bill, longer legs, larger body size and paler overall plumage. It also exhibits behavioural traits that are different from those of arboreal tits, as it forages on the ground and digs burrows or tunnels for roosting and nesting [6] . In all these characters, the ground tit closely resembles ground jays of the genus Podoces in the family Corvidae (crows, jays, magpies and their allies). Indeed, the ground tit was long considered to be the smallest member of Corvidae and placed in a monotypic genus ( Pseudopodoces ). Given that both ground jays and ground tit exclusively dwell in high steppes and adapt to living on the ground, their morphological similarities are likely to result from convergent evolution [7] , for example, long decurved beaks for probing the ground, elongated legs for hopping locomotion and large body size for heat retention. The most severe environmental challenges to the ground tit in the Tibetan plateau are the hypoxic and low temperature. It can thus be hypothesized that this species has increased energy metabolism rates and elevated responses to hypoxic conditions, as have been shown for Tibetan native people and the yak [8] , [9] , [10] . To test this, we have generated and analysed the genome of the ground tit and re-sequenced the genome of two closely related tits, the great tit, Parus major and the yellow-cheeked tit, P. spilonotus , and the Mongolian ground jay, Podoces hendersoni . Our results show that the ground tit exhibits elevated responses to hypoxia and increased energy metabolism, the same survival strategies that have been previously shown in other high-altitude animals. Our study also suggests other adaptations in the ground tit to a life at high altitudes (for example, increased skeletal development, reduced feather keratins and olfactory genes). This genomic study provides insights into both genetic modifications that are crucial to a life in this extreme alpine environment, as well as some unexpected genomic consequences resulting from these adaptations. Genome assembly and annotation We sequenced the genome of a female ground tit from Gahai, Gansu, China ( Fig. 1 ) using a whole-genome shotgun strategy and the Illumina HiSeq 2000 platform. De novo assembly of 1.85 billion reads from five paired-end and mate-pair libraries provides 171-fold coverage with a total assembly length of 1080.6 Mb ( Supplementary Table S1 ), which approximates the genome size estimated using K-mer frequency method ( Supplementary Table S2 and Supplementary Fig. S1 ). The contig and scaffold N50 sizes are 88.3 and 1615.4 kbp, respectively, with the largest scaffold spanning 6961.4 kbp and gap regions accounting for 0.85% of the whole assembly ( Supplementary Table S3 ). The genome assembly covered 99.63% of the 11,453 high-quality unigenes assembled from 23.74 Gb RNA sequence data for lung and muscle tissues ( Supplementary Tables S1–S4 ). Of unigenes that were covered by genome sequences, 89.19% exist in one intact scaffold, ensuring that the assembly covered most of the transcriptional regions. The high overall coverage of 99.6% ( Supplementary Fig. S2 ) and similarly comparable size and composition to other bird genomes ( Supplementary Table S5 and Supplementary Fig. S3 ) indicate that the assembly of the ground tit genome is characterized by a high level of accuracy. 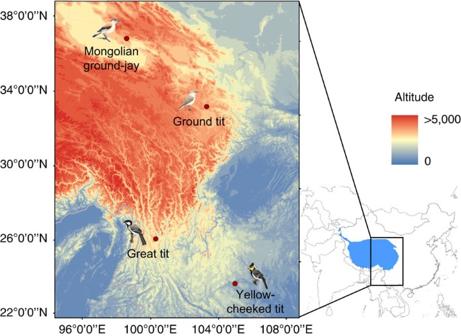Figure 1: Sampling localities of three tits and the ground jay. The ground tit was collected in Gahai, Gansu province, China; the yellow-cheeked tit in Longlin, Guangxi province, China; the great tit in Lijiang, Yunnan province, China; and Mongolian ground jay in Delingha, Qinghai province, China. Figure 1: Sampling localities of three tits and the ground jay. The ground tit was collected in Gahai, Gansu province, China; the yellow-cheeked tit in Longlin, Guangxi province, China; the great tit in Lijiang, Yunnan province, China; and Mongolian ground jay in Delingha, Qinghai province, China. Full size image By genome-wide searching and homology prediction against the Repbase database, we show that 9.09% of the ground tit genome belongs to the transposable element (TE) families ( Supplementary Table S6 ). The overall repeat content, especially DNA transponsons (0.37%), long interspersed nuclear element (3.67%) and long terminal repeats (3.03%), is similar to that of zebra finch (0.26%, 3.40% and 3.55%, respectively), but differed from that of chicken (0.97%, 6.29% and 1.49%) ( Supplementary Table S7 ). There is a large proportion of highly divergent repeats compared with other avian genomes ( Supplementary Fig. S4 ), suggesting considerable ancient transposition with little recent activity. After masking the repetitive regions, we annotated the genes using a combinational method based on homology search, ab initio prediction, publicly available EST/cDNA evidences and direct mRNA sequencing evidences ( Supplementary Table S8 ). This generated a total of 17,520 protein-coding genes and 830 other RNA genes ( Supplementary Tables S9 and S10 ). Of the protein-coding genes, 86.94% have homologues in the protein databases (including Swissprot and TrEMBL), and were classified into functional categories according to InterPro (ref. 11 ), KEGG (ref. 12 ) pathway database and Gene Ontology (GO) (ref. 13 ) ( Supplementary Table S11 ). The ground tit is a real tit and not a jay To further test the phylogenetic position of the ground tit based on whole-genomic sequence, we re-sequenced one great tit, one yellow-cheeked tit and one Mongolian ground jay to ~10-fold sequence coverage using Illumina technology, and aligned the data to the ground tit genome. The whole-genome alignment confirmed that the ground tit is much more closely related to the other tits than to the ground jay; the re-sequencing data of the two tit species mapped to 78–80% of the ground tit genome, and to only 9.7% of ground jay ( Fig. 2a and Supplementary Table S12 ). The phylogenetic reconstruction clearly supports the grouping of the ground tit with the other two tit species ( Fig. 2c ). The estimated time of divergence between the ground tit and the other tits is between 7.7 and 9.9 million years ago. 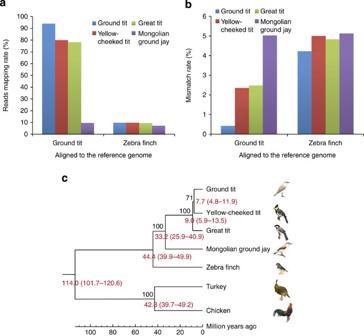Figure 2: Phylogenetic relationship and distance of the ground tit. (a) Percentage of sequencing reads of the ground tit, great tit, yellow-cheeked tit and Mongolian ground jay mappable to either the ground tit or the zebra finch genomes. (b) Mismatch rate between the reads and the subject genome among the mappable reads. (c) Phylogenetic tree based on 68 single-copy ortholog genes suggests that the ground tit is more closerly related to the great tit and the yellow-cheeked tit than to the ground jay. The divergence time is given in millions of years in red colour. The bootstrap values are shown above the nodes. The relative rates of molecular evolution are expressed as the branch lengths. Estimates of divergence times (millions of years) calculated from the rate of sequence similarity are indicated at each node. Figure 2: Phylogenetic relationship and distance of the ground tit. ( a ) Percentage of sequencing reads of the ground tit, great tit, yellow-cheeked tit and Mongolian ground jay mappable to either the ground tit or the zebra finch genomes. ( b ) Mismatch rate between the reads and the subject genome among the mappable reads. ( c ) Phylogenetic tree based on 68 single-copy ortholog genes suggests that the ground tit is more closerly related to the great tit and the yellow-cheeked tit than to the ground jay. The divergence time is given in millions of years in red colour. The bootstrap values are shown above the nodes. The relative rates of molecular evolution are expressed as the branch lengths. Estimates of divergence times (millions of years) calculated from the rate of sequence similarity are indicated at each node. Full size image Evolution of gene families By comparing the protein sequences of the ground tit to the annotated protein sequences of other available avian species, we identified 9,056 ground tit genes in 8,479 families common to these avian taxa ( Fig. 3b and Supplementary Table S13 ). We classified 8,095 single-copy genes and 981 multiple-copy genes in the ground tit genome ( Supplementary Table S14 ). Sequence depth of these multiple-copy genes was in the same range as for single-copy genes ( Supplementary Fig. S5 ). The ground tit genome contained 1,516 unique genes (8.65%), which were mainly enriched in two categories: biological process and energy metabolism ( Supplementary Table S15 ). In addition, 55 gene families were significantly expanded and 10 contracted in the ground tit ( Fig. 3a ), which were over-represented in energy metabolism and immunity, respectively ( Supplementary Table S16 ). Gene loss enrichment analysis showed that the ground tit has lost many genes related to olfactory perception and feather keratins ( Supplementary Table S17 ). Subsequently, 7,190 high-confident 1:1:1:1 orthologous genes were identified in the ground tit, zebra finch, chicken and turkey ( Fig. 3b ). Estimates of non-synonymous to synonymous substitution rates ( Ka / Ks ) based on these orthologous genes are shown in Supplementary Fig. S6 . We identified 2,051 positively selected genes in the ground tit genome and these genes were enriched in energy metabolism and response to hypoxia ( Supplementary Table S18 ). 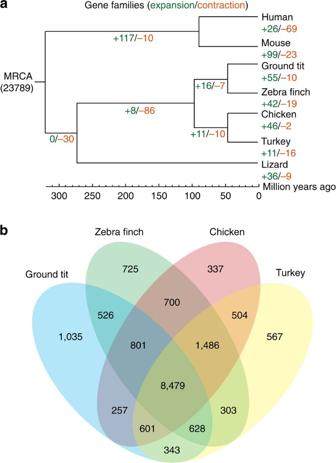Figure 3: Comparison of gene families. (a) Gene family expansion and contraction in each evolutionary branch. The numbers of expanded (blue) and contracted (red) gene families are shown at the nodes in the phylogenetic tree and under the names of the organisms. MRCA: most recent common ancestor. The divergence time is given in millions of years. It shows that 55 and 10 gene families are expanded and contracted in the ground tit, respectively. (b) A Venndiagram of predicted gene families in ground tit, zebra finch, chicken and turkey. The number of unique or shared gene families is listed in each diagram component. Figure 3: Comparison of gene families. ( a ) Gene family expansion and contraction in each evolutionary branch. The numbers of expanded (blue) and contracted (red) gene families are shown at the nodes in the phylogenetic tree and under the names of the organisms. MRCA: most recent common ancestor. The divergence time is given in millions of years. It shows that 55 and 10 gene families are expanded and contracted in the ground tit, respectively. ( b ) A Venndiagram of predicted gene families in ground tit, zebra finch, chicken and turkey. The number of unique or shared gene families is listed in each diagram component. Full size image We further reconstructed genomic sequences of the common ancestor of the ground tit, yellow-cheeked tit and great tit, and calculated and compared the Ka / Ks ratios of these three tits. To generate comparable databases among the three tits, we retained only sequences that mapped 100% with the ground tit’s exons, resulting in a total of 11,161 (63.7%) and 10,396 genes (59.3%) for the yellow-cheeked tit and the great tit, respectively. Ka / Ks analyses revealed that genes regulating energy metabolism, hypoxia response and skeletal development evolve at higher rates in the ground tit than in two other species ( Supplementary Table S19 ). Elevated energy metabolism and response to hypoxia Four lines of evidence support that ground tit has increased energy metabolism rate and elevated response to hypoxic condition. First, 10 of the 18 enriched GO categories in ground tit-specific genes are related to metabolism ( Supplementary Table S15 ). Second, gene families involved in energy metabolism are substantially expanded in the ground tit genome, supported by 8 out of the 15 enriched GO categories ( Supplementary Table S16 ). Third, signatures of positive selection in ground tit genes are significantly enriched for energy metabolism and hypoxia response (7 of the 12 categories, Supplementary Table S18 ). Fourth, more than half of GO terms enriched by elevated Ka / Ks ratios are related to energy metabolism and hypoxia response ( Supplementary Table S19 ). The capacity for sustained thermogenesis is critical for survival under cold stress conditions. We observed many positively selected and lineage-specific genes of the ground tit in fatty-acid metabolism pathways ( Fig. 4 ). These pathways are related to functions from fatty-acid anabolism to catabolism, and are associated with disorders of fatty-acid oxidation and peroxisomal β-oxidation enzyme deficiency. 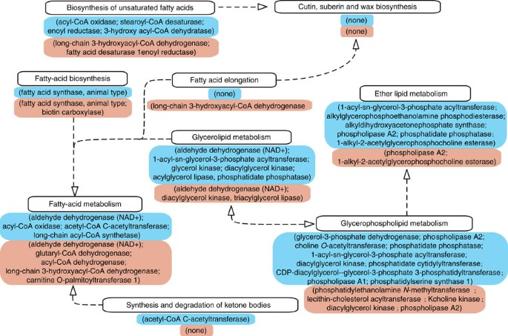Figure 4: Selection in fatty-acid metabolism pathways. Postively selected and lineage-specific genes are indicated in blue and red, respectively, under each pathway of the ground tit. Annotations and connections are presented in accordance with KEGG standards, where dashed lines represent indirect relationships. Figure 4: Selection in fatty-acid metabolism pathways. Postively selected and lineage-specific genes are indicated in blue and red, respectively, under each pathway of the ground tit. Annotations and connections are presented in accordance with KEGG standards, where dashed lines represent indirect relationships. Full size image Some genes related to hypoxia response showed signals of positive selection in the ground tit ( Table 1 ). Four of these, the HIF1AN , ANGP4 , ADAM9 and MDH1B , are previously shown to be under positive selection in the Tibetan yak and in human populations living at high altitudes in Tibet, Andes and Ethiopia, indicating their probable role in the adaptation to high altitudes [10] , [14] , [15] , [16] . HIF1AN is known as HIF-1 α-subunit inhibitor and ANGP4 is a member of the angiopoietin family and involved in the remodelling, maturation and stabilization of the vascular network [10] , [14] . ADAM9 is an important regulator of HIF-1 α (ref. 14 ). These three genes are part of the hypoxia-inducible pathway and directly involved in angiogenesis, vasodilatation and energy metabolism in response to hypoxia [10] , [14] , [15] . In addition we also found a few other positively selected genes that may be involved in response to hypoxia. SRF , TXNRD2 and WNT7B regulate the vasculogenesis in lung and heart, and are important mediators in hypoxia-induced angiogenesis [17] , [18] , [19] . MTOR and PSMD2 are involved in protein synthesis and cellular response under oxidative stress [20] , [21] . Hypoxia-induced experiments in both laboratory and at high altitudes have confirmed the role of these genes directly in oxidative stress [17] , [18] , [19] , [20] , [21] . Table 1 Positively selected genes involved in hypoxia response. Full size table Gene loss related to the immune system Long-term exposure to hypoxia in high altitudes is known to suppress immune responses in people living in Nepal and Himalayas [22] , and other high-altitude environments [23] . Immunity may also be affected by exposure to ultraviolet (UV) radiation. UV exposure in laboratory affects antigen presentation, inflammatory response and cytokine production [24] , [25] . Hypoxia and strong UV radiation may have shaped the ground tit genome, in which 6 out 10 gene families have lost genes involved in the immune system, for example, immune response, major histocompatibility complex (MHC) protein complex, antigen processing and chemokine activity ( Table 2 and Supplementary Table S20 ). Table 2 Different gene families among four bird genomes. Full size table Loss of olfactory receptor genes Comparative genomic study suggested that ecological selective pressures such as habitat and diet have driven the evolution of avian olfaction [26] . The total number of olfactory receptor genes in a genome reflects how many different scents can be detected and distinguished [27] , [28] . For example, a decline in proportion of olfactory receptor genes in a specialist bird, the snow petrel ( Pagodroma nivea ), has been suggested to be associated with a less keen sense of smell when compared with two generalists, the kiwi ( Apteryx australis ) and the kakapo ( Strigops habroptilus ) [26] . As the ground tit inhabits a cold and dry plateau dominated by arid alpine meadow, it may be postulated that its olfactory system has become less sensitive to scents, and indeed, the number of olfactory receptor genes is very low in the ground tit ( Table 2 and Supplementary Table S21 ). Skeletal development and feather β-keratin We detected an increased rate of evolution in genes related to skeletal development in the ground tit ( Supplementary Table S19 ). In addition we found positively selected and ground tit-specific genes involved in bone morphogenesis ( Supplementary Table S22 ). Enrichment of these genes identified two pathways: BMP transforming growth factor-β signalling pathway and its downstream pathway, MAP kinase pathway ( Fig. 5 ). The BMP transforming growth factor has a central role in the skeletal development and has important implications in the formation of claws and bill in birds [29] , [30] . These positive and lineage-specific genes identified in the BMP pathway are mostly transmembrane receptors, which activate the downstream SMAD-dependent and/or MAP kinase pathways by the oligomerization of the BMP receptors. Both pathways regulate the transcription of specific target genes that are involved in bone formation [30] . Recent studies have suggested that the mutations in BMPR I gene affect the cartilage formation in humans, and the limb development in chicken [31] . Alterations of these genes in the BMP signalling pathways may affect the growth of the skeletal components of the ground tit, but this needs to be validated by future functional assessments of these genes. 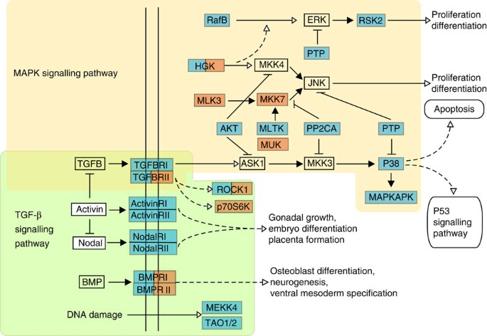Figure 5: Genes involved in the BMP and MAP kinase pathways. We identified positively selected genes (indicated in blue) and lineage-specific genes (red) that fall within BMPs signalling pathway in the TGF-β family members (KEGG: 04350), together within MAP kinase pathway (adapted from KEGG pathway 04350 and 04010). Abbreviations, annotations and connections are presented in accordance with KEGG standards: solid lines represent direct relationships between enzymes (boxes) and metabolites (circular nodes), dashed lines indirect relationships, arrowheads denote directionality, the double vertical lines indicate cell membrane, with the left being extracellular and right intracellular region. Figure 5: Genes involved in the BMP and MAP kinase pathways. We identified positively selected genes (indicated in blue) and lineage-specific genes (red) that fall within BMPs signalling pathway in the TGF-β family members (KEGG: 04350), together within MAP kinase pathway (adapted from KEGG pathway 04350 and 04010). Abbreviations, annotations and connections are presented in accordance with KEGG standards: solid lines represent direct relationships between enzymes (boxes) and metabolites (circular nodes), dashed lines indirect relationships, arrowheads denote directionality, the double vertical lines indicate cell membrane, with the left being extracellular and right intracellular region. Full size image The ground tit spends most of its time on the ground and the observed reduction of feather β-keratin genes may reflect this. Avian feather β-keratin genes encode proteins vital for the formation of feathers, and recent biophysical studies have demonstrated the role of β-keratin genes in forming the elasticity of the feather [32] . Cameron et al. [33] found that birds capable of flight generally have a higher β-keratin composition in their feathers than flightless birds. Weiss and Kirchner [34] have provided a hierarchical model of feather β-keratins and associated matrices to explain the variable plasticity of feathers and proposed that feather β-keratin genes may have gone through numerous duplication events to allow for greater diversity of feathers both in function and form, including powered flight. The ground tit was long considered to belong to the crow family and placed in monotypic genus Pseudopodoces , which was supposed to be closely related to the ground jays [4] . It was later shown that the ground tit, instead of being the world’s smallest corvid, is the world’s largest tit. Our genomic study further confirms this taxonomic conclusion. The ancestor of the ground tit split off from other tits between 7.7 and 9.9 million years ago. Although the uplift of the Tibetan plateau started already around 50 million years ago, a significant increase in altitude occurred about 8–10 million years ago [35] . It seems plausible that the formation of the extremely arid and cold conditions of the Tibetan plateau drove speciation of the ground tit. The ground tit genome can be characterized by its adaptations to the extreme living conditions of the high-altitude habitat on the Tibetan plateau. One major adaptation is an increased evolutionary rate and positive selection on genes involved in hypoxia response and energy metabolism, analogous to those observed in other organisms in Tibet [10] , [14] , [15] , [16] , the Andes and other high-altitude environments [17] , [18] , [19] . Interestingly, most genes involved in increased energy metabolism are related to fatty-acid metabolism pathways. A previous study has demonstrated that an enhanced capacity of fatty-acid metabolism in the high-altitude deer mice ( Peromyscus maniculatus ) [16] . Similarly, studies of birds in the Arctic and at high altitudes have shown that lipids have a crucial role in regulatory thermogenesis by acting both as substrates for and activators of thermogenic processes [8] , [9] . Relative to the oxidation of carbohydrates, the oxidation of lipids has a higher energy density [16] and can elevate the thermogenic capacity for a prolonged period [9] . The strong selection in lipid metabolism may have been developed as an optimal fuel-use strategy for the ground tit that is forced to cope with the challenge for chronic cold stress conditions. Another adaptation to a life on the Tibetan plateau may be the loss of many immune genes, many of which are associated with MHC-mediated antigen recognition and processing. MHC is a group of cell surface receptors that function to present antigen to T cells responsible for cell-mediated immune responses. Upon non-self recognition, the antigen-presenting cell will be eliminated. This process forms the basis of cellular immune defence against pathogens, including viruses and bacteria [36] . The diversification and multitude of pathogens have been used to explain the diversity of MHC genes, and changes of MHC genes have an integral role in immune innovation in birds [37] . It is possible that the reduction of MHC genes in the ground tit is due to a lighter load of microorganisms present in the Tibetan plateau and therefore a decreased risk of opportunistic infections [38] . The loss of olfactory receptor genes may be a third adaptation if it proves to be related to the limited variety of scents in the arid, alpine meadow environment. However, ecological adaptation alone may not explain the loss of olfactory receptor genes in the ground tit. For example, when comparing the genome of the yak, a species that also inhabits the Tibetan Plateau, to that of domestic cattle, an increased number of olfactory receptor genes were found in the yak [14] . The explanation of the loss of olfactory receptor genes in the ground tit must await comparisons with genomes of closely related species inhabiting lower altitudes. A fourth adaptation to a life in arid conditions above the tree line is an increased evolutionary rate in skeletal development genes and a reduced number of feather keratin genes. In the ground tit these changes in the genome may be expressed in the longer decurved bill, longer legs, larger body size and less developed flying capability compared with other tits. Unlike the ground tit’s arboreal ancestor that used tree holes for nesting, the ground tit lives above the tree line and has developed the ability to dig burrows for roosting and nesting [5] . Adaptations to a life on the ground are likely to impose a selective constraint on skeletal development. In addition the ground tit is the only species of Parus that has lost its skeletal pneumatic openings in the pneumotricipital fossa of the humerus. The loss of the pneumotricipital fossa is commonly observed in birds that are ground living and that only rarely fly and is explained to be caused by a relaxation of selection for extensive air sacs and diverticula [5] . The role of genes controlling skeletal development and feather β-keratin genes in high-altitude adaptation has not been reported before. Further functional studies and expression profiles of these genes are needed to better understand how these genes are involved in the morphological changes of the ground tit. The similarities in external morphology of the ground tit and the ground jays should be considered as the results of convergently evolved adaptations to a life in an arid environment above the tree line. To our knowledge this is the first attempt to identify the genomic basis of adaptations leading to this morphology. The genomic study of the ground tit provides new understanding of the unique adaptations to a high-altitude environment (for example, increased skeletal development, reduced feather keratins and olfactory genes), in addition to other strategies for survival (for example, response to hypoxia, increased energy metabolism) known from other high-altitude species. Comparisons of genomes from closely related species inhabiting high altitudes and lowland environments, respectively, are needed to further explore the genetic foundation for these adaptations. Sample information The female ground tit was collected by mist net in Gahai, Gansu province of China, at an elevation of 3,500 m. The great tit was collected in Lijiang, Yunnan province of China and the yellow-cheeked tit in Jinzhongshan Natural Park, Guangxi province of China. The Mongolian ground jay was collected from Delingha, Qinghai province of China ( Fig. 1 ). The tissues of these birds were stored in liquid nitrogen and transported to the sequencing center. The specimens were collected with permission from the Forestry Department of China and conform to the National Wildlife Conservation Law in China. Tissue collection procedures also conform to the regulations of the animal experimental and medical ethics committee of the Institute of Zoology, Chinese Academy of Sciences. The Zoological Museum of Institute of Zoology has the authority for specimen collecting and exemption of export/import of samples for scientific purposes (No. 1999/84, provided by Article VII from CITES). Sequencing and assembly DNA was isolated from the liver using the Qiagen DNeasy Blood and Tissue Kit under the protocol provided by the manufacturer. Short-insert-sized (180 and 500 bp) and mate-pair (2, 5 and 10 kb) DNA libraries were constructed for the ground tit and 500 bp insert-sized libraries were constructed for the yellow-cheeked tit, the great tit, and the Mongolian ground jay. RNA was extracted from lung and muscle tissue and RNA sequencing libraries were constructed using the Illumina mRNA-Seq Prep Kit. All the libraries were sequenced on the Illumina HiSeq 2000 platform in paired-end form. After filtering out low quality and clonally duplicated reads, a total of 185.18-Gb DNA (171x) was obtained for de novo assembly of the ground tit genome, and 23.74-Gb RNA sequence data for gene annotation. Paired-end sequence data from the genomic DNA libraries were assembled using short oligonucleotide analysis package SOAP denovo [39] . Assembly quality and completeness were assessed by checking all read pair coverage and supporting evidence. The final contig and scaffold sizes, N50 and N90, were calculated based on the minimum length of sequence of >100 bp. The sequencing coverage, depth, GC content distribution and heterozygosity rate of the assembled genome sequence were evaluated by mapping all sequencing reads of the short-insert-sized libraries back to the scaffolds using BWA [40] . Genome annotation We searched for tandem repeats across the genome of the ground tit using the software Tandem Repeats Finder. TEs were predicted in the genome by homology search against the known TE sequences in RepBase (RM database version 20110920) using RepeatMasker and RepeatProteinMask [41] with default parameters. To make the ground tit genome comparable to the other vertebrate genomes included in the analysis, we employed the same pipeline and parameters to re-run the repeat annotation in human, rat, chicken and zebra finch genomes. The diversity rate of the detected TEs was calculated by comparison of the annotated TE copies to the consensus sequences derived from Repbase. We used homology, ab initio prediction, EST and RNA sequence to identify protein-coding genes. For homology-based gene prediction, human, rat, zebra finch, chicken and turkey proteins were downloaded from Ensembl Release 67 ( http://www.ensembl.org/info/data/ftp/index.html ) and mapped onto the repeat-masked ground tit genome using TBLASTN [42] . In next step, homologous genome sequences were aligned against the matching proteins using Genewise [43] to define gene models. Subsequently, we used the ab initio gene prediction, Genscan [44] and Augustus [45] to predict protein-coding genes using parameters trained from a set of high-quality homologue prediction proteins. Finally, RNA sequence data were mapped to genome using TopHat [46] , and transcription-based gene structures were obtained by Cufflinks. The structures and EST sequence were mapped to the genome by Genewise [43] . The final gene set was generated by merging all genes predicted by the three methods using EvidenceModeler [47] , and removed all genes with length shorter than 50 amino acids and only with ab initio support and FPKM confidence <5. By this we obtained a reference gene set that contained 17,520 genes. Gene functions were assigned according to the best match of the alignment to the SwissProt and Translated EMBL Nucleotide Sequence Data Library databases [48] using BLASTP. We annotated motifs and domains using InterProScan by searching publicly available databases, including PFAM, PRINTS, PROSITE, PRODOM and SMART. We used GO to describe gene products, and GO IDs for genes were obtained from the corresponding InterPro entry. We also mapped the ground tit reference genes to KEGG pathway databases and identified the best match for each gene. Phylogeny reconstruction We generated about 12-Gb sequences for each of the yellow-cheeked tit, the great tit and the Mongolian ground jay. We aligned the high-quality reads of these birds (average quality larger than 20) to the ground tit genome using SOAP2. The ground tit genome was provided as a reference to define homologous genes in the three re-sequenced birds using TBLASTN and Genewise. Only a total of 68 single-copy gene families were defined because of 9.7% mapping rate of Mongolian ground jay reads to the ground tit genome. The phylogenetic relationship among these four species was inferred by maximum likelihood analysis based on the Tamura-Nei model, with zebra finch, turkey and chicken as the outgroups. The protein sequences of the 68 single-copy gene families were aligned using MUSCLE [49] , and then converted to the corresponding nucleotide sequence alignment. MODELTEST [50] was used to select the best substitution model (GTR+gamma+I) and Treebest [51] used to reconstruct the phylogenetic tree. Bootstrap support for internal branches was evaluated from 1,000 full-heuristic searches. Divergence times between species were calculated using MCMC tree program implemented in the PAML (ref. 52 ). Gene family To define gene families that descended from a single gene in the last common ancestor, we downloaded all protein-coding genes of zebra finch, chicken, turkey and lizard from Ensembl Release 67. The longest translation form was chosen to represent each gene. Treefam [53] methodology was used to define gene families. To identify gene family evolution as a stochastic birth and death process, where gene family either expands or contracts per gene per million years independently along each branch of the phylogenetic tree, we applied the likelihood model originally implemented in the software package Café [54] . The phylogenetic tree topology and branch lengths were taken into account to infer the significance of change in gene family size in each branch. The gene families of the ground tit were compared with those of other genomes, and significant levels of expansion and contraction were determined at 0.05. Positively selected genes To detect genes evolving under positive selection in the ground tit, we identified 7,190 high-confident 1:1:1:1 orthologous genes in the ground tit, zebra finch, chicken and turkey ( Fig. 3b ). The optimized branch-site model of codon evolution was used, in which likelihood ratio test P -values were computed assuming that a null distribution was a 50:50 mixture of a χ 2 distribution with one degree of freedom and a point mass at zero. Fisher’s exact tests were used to test for over-represented among functional categories in GO and IPR. Multiple tests were done by using FDR (false discovery rate) correction to adjust the P -value (cutoff: 0.05). Ka/Ks analysis between ground tit and other tits We used PAML to infer the ancestral sequences (the most recent common ancestor between the ground tit and yellow-cheeked tit/great tit). We used the Yang-Nielsen model to calculate Ka and Ks values for each pair of species (ground tit, zebra finch, chicken, turkey). The numbers and ratios of non-synonymous and synonymous substitutions ω ( Ka / Ks ) in each branch were estimated using Codeml with the F3 × 4 codon frequency model (which calculates codon frequencies using base composition at the three codon positions) and different ω ratios across branches and a single ω ratio across sites, and separate estimation of κ per gene. To explore the evolution of function catalogue, we use the GO annotation of the ground tit. Only the GO catalogues containing no <20 genes were selected for further analysis. Ka / Ks ratio between the ground tit and its ancestor was used to estimate rapidly evolving function categories. The binomial test was used to identify GO categories. All P -values were adjusted for multiple comparisons by the Bonferroni method. Accession codes Sequencing data for the ground tit, the yellow-cheeked tit, the great tit and the Mongolian ground jay have been deposited in Short Read Archive under project number PRJNA 179234 and accession code SRA061431. RNA sequence and RPKM files have been deposited in Gene Expression Omnibus under accession code GSE44779. How to cite this article: Qu, Y. et al. Ground tit genome reveals avian adaptation to living at high altitudes in the Tibetan plateau. Nat. Commun. 4:2071 doi: 10.1038/ncomms3071 (2013).